The metastasis-promoting S100A4 protein confers neuroprotection in brain injury Identification of novel pro-survival factors in the brain is paramount for developing neuroprotective therapies. The multifunctional S100 family proteins have important roles in many human diseases and are also upregulated by brain injury. However, S100 functions in the nervous system remain unclear. Here we show that the S100A4 protein, mostly studied in cancer, is overexpressed in the damaged human and rodent brain and released from stressed astrocytes. Genetic deletion of S100A4 exacerbates neuronal loss after brain trauma or excitotoxicity, increasing oxidative cell damage and downregulating the neuroprotective protein metallothionein I+II. We identify two neurotrophic motifs in S100A4 and show that these motifs are neuroprotective in animal models of brain trauma. Finally, we find that S100A4 rescues neurons via the Janus kinase/STAT pathway and, partially, the interleukin-10 receptor. Our data introduce S100A4 as a therapeutic target in neurodegeneration, and raise the entire S100 family as a potentially important factor in central nervous system injury. Brain injury is a complex process with a primary damage that triggers inflammatory and apoptotic pathways leading to delayed neuronal death. This secondary damage, observed in major neurological disorders, such as brain trauma, epilepsy, ischaemia or stroke, is a key factor defining the outcome [1] . The delayed neurodegeneration is accompanied by upregulation of many brain proteins, some of which may be crucial for neuronal survival; however, for most of them, the function remains unknown. Similar uncertainty exists for the multifunctional S100 protein family, which is implicated in multiple human diseases by regulating apoptosis, inflammation and cell motility and proliferation [2] , [3] . At least 12 S100 proteins are expressed in the nervous system during neurodegeneration and neuronal plasticity [4] , [5] , [6] , but only S100B and S100A10 have to date been linked to brain pathologies [7] , [8] . For S100B and S100A12, the receptor for advanced glycation end products (RAGE) was identified in inflammatory and neural cells conferring both trophic and deleterious effects depending on extracellular S100 levels [9] . However, many biological functions of S100 proteins are RAGE-independent [2] , suggesting the existence of yet unknown targets and roles for the S100 family. S100A4 (Mts1) is a small Ca 2+ -binding protein expressed as homodimer (22 kDa), but oligomerized in the presence of Ca 2+ and/or under non-reducing conditions [10] , [11] . Initially, it was identified as a metastasis promoter and mainly studied in relation to cancer [2] , [10] . Although S100A4 is not tumorigenic per se , it promotes motility and invasion of already existing tumour cells, resulting in aggressive metastasis. This makes S100A4 a major prognostic marker in many cancer types [12] . Intracellularly, S100A4 binds to several targets regulating cytoskeletal dynamics and cell motility and proliferation [10] , [13] . Moreover, S100A4 is secreted from both tumour [13] , [14] and non-malignant [15] cells, and exerts extracellular effects regulating, in particular, angiogenesis [16] , cell migration and cardiomyocyte differentiation and hypertrophy [17] . Signalling by extracellular S100A4 is not yet well characterized and presumably involves both a common S100 target RAGE and other, yet unidentified receptors [18] . In our previous studies, we have demonstrated that extracellular S100A4 acts as a neuritogenic factor in cultured neurons activating several signalling pathways and likely functioning via multiple receptors independently of RAGE [11] , [19] . Interestingly, S100A4 is also expressed in white matter (WM) astrocytes and myelinated tracts of the intact rat central nervous system (CNS) [20] , and traumatic brain injury (TBI) in rodents induces marked upregulation of both the S100A4 gene [21] and protein [22] . However, the function of S100A4 in the nervous system remains unclear. Here we identify a novel neuroprotective role for S100A4 using in vivo models of major brain pathologies, TBI and excitotoxicity, in S100A4-deficient mice. Moreover, we explore the mechanism of S100A4-induced neuroprotection, identify neurotrophic motifs in S100A4 and show that synthetic peptides encompassing these motifs have therapeutic potential for treatment of neurological disorders. S100A4 is upregulated in brain injury and protects neurons Because S100A4 upregulation has to date only been shown in rodents, we first analysed S100A4 expression in the human brain [14] . In pericontusional biopsies from patients with cortical brain trauma, S100A4 was readily detectable in WM astrocytes (4.9±1.8 × 10 5 cells mm −2 , n =6) and in blood cells, previously known to express S100A4 (ref. 23 ), whereas it was absent in the WM and cortex of intact brains ( Fig. 1a , Supplementary Table S1 ). To address the S100A4 expression in mice after TBI we used a cryogenic lesion, which is a closed brain injury producing a secondary response similar to that seen after severe head trauma [24] , [25] . Similarly, S100A4 was only detected in the injured animals in WM and blood cells at the lesion site ( Fig. 1b , S100A4-specific antibodies characterized in El Naaman et al . [26] and Supplementary Fig. S1a ,b). Interestingly, S100A4 was also induced in the contralateral WM, most probably following the spreading astrocytic activation, which occurs in focal brain injuries [27] , [28] and was also observed in this model (glial acidic fibrillary protein (GFAP) staining, Supplementary Fig. S1c ). To test whether the S100A4 expression pattern was related to the trauma type, we examined S100A4 distribution after kainic acid (KA)-evoked excitotoxicity, a diffuse brain injury used as a model of human temporal lobe epilepsy [29] , [30] . Here S100A4 was induced not only in the WM, but also in the hippocampus, a region most vulnerable to excitotoxicity ( Fig. 1b , KA). Thus, in both humans and mice, S100A4 was upregulated in the brain areas affected by damage indicating its role in post-traumatic brain plasticity. To test whether S100A4 could be released from activated or lysed S100A4-expressing cells, we subjected cultured early postnatal hippocampal astrocytes to hydrogen peroxide (H 2 O 2 ), an inducer of oxidative stress, contributing to many brain insults [31] . Despite robust cytoplasmic expression of S100A4, no detectable S100A4 release from untreated cells was observed ( Fig. 1d ). However, already 2 h after H 2 O 2 treatment, S100A4 was readily detected in the extracellular medium ( Fig. 1d ). At 24 h, some of the cultures subjected to a high H 2 O 2 concentration (160 μM), also exhibited decreased cell counts (70–85% of untreated, Fig. 1d , ‘damaged’). In these cultures, the amount of released S100A4 was ca five-fold higher ( Fig. 1d ), suggesting that even minor astrocytic damage can result in a significant increase of extracellular S100A4. 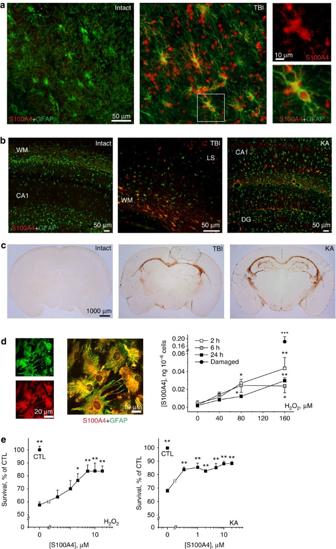Figure 1: S100A4 is upregulated in the injured brain and protects neuronsin vitro. (a) S100A4 is induced in the human brain following TBI. S100A4/GFAP stainings of intact (n=3) and injured (TBI,n=6) human brains (WM). (Inset) S100A4-expressing astrocyte, magnified. (b,c) S100A4 expression in the mouse brain following TBI (72 h post injury,n=8) or KA-induced excitotoxicity (48 h post injury,n=8). LS, lesion site; DG, dentate gyrus. (d) S100A4 is released from astrocytes subjected to oxidative stressin vitro. ANOVA versus untreated cultures, five to seven independent experiments. (e) S100A4 is neuroprotectivein vitro. CTL, neuronal viability in untreated controls. ANOVA versus cultures treated with H2O2or KA only, five independent experiments. Results are expressed as means±s.e.m. *P<0.05; **P<0.01; ***P<0.001. Scale bars, 50 μm (a,b), 10 μm (a, inset;d), 20 μm (d, inset), 1,000 μm (c). Figure 1: S100A4 is upregulated in the injured brain and protects neurons in vitro . ( a ) S100A4 is induced in the human brain following TBI. S100A4/GFAP stainings of intact ( n =3) and injured (TBI, n =6) human brains (WM). (Inset) S100A4-expressing astrocyte, magnified. ( b , c ) S100A4 expression in the mouse brain following TBI (72 h post injury, n =8) or KA-induced excitotoxicity (48 h post injury, n =8). LS, lesion site; DG, dentate gyrus. ( d ) S100A4 is released from astrocytes subjected to oxidative stress in vitro . ANOVA versus untreated cultures, five to seven independent experiments. ( e ) S100A4 is neuroprotective in vitro . CTL, neuronal viability in untreated controls. ANOVA versus cultures treated with H 2 O 2 or KA only, five independent experiments. Results are expressed as means±s.e.m. * P <0.05; ** P <0.01; *** P <0.001. Scale bars, 50 μm ( a , b ), 10 μm ( a , inset; d ), 20 μm ( d , inset), 1,000 μm ( c ). Full size image We next evaluated how extracellular S100A4 affects neuronal survival using two physiologically relevant in vitro models of brain injury. Neuronal death was triggered either by H 2 O 2 or by an excitotoxic agent KA. Extracellular S100A4 rescued neurons in both models, and this effect did not diminish or reverse at higher protein concentrations ( Fig. 1e ) indicating a neuroprotective function for S100A4. Genetic deletion of S100A4 impairs neuroprotection We then asked whether S100A4 deficiency aggravates brain damage. In mice subjected to TBI, a well-defined cortical lesion was present, which caused neuronal death in the surrounding area ( Fig. 2a , left, wild-type (WT)). Remarkably, the number of apoptotic neurons was ~70% higher in the S100A4 −/− than in WT animals ( Fig. 2a , cell identity confirmed by the neuronal marker NeuN/TdT-mediated dUTP nick end labelling co-staining, Supplementary Fig. S1d ). Moreover, consistent with the S100A4 ability to protect neurons against the oxidant-caused death in vitro , the S100A4 −/− mice had strongly increased susceptibility to oxidative stress after TBI ( Fig. 2b ). 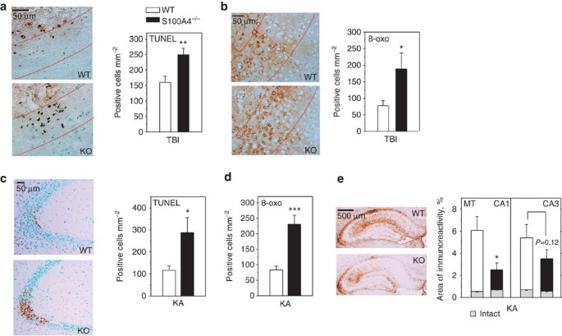Figure 2: S100A4 deficiency exacerbates brain injury. (a,b) Neuronal death (TdT-mediated dUTP nick end labeling (TUNEL),a) and oxidative stress (8-oxoguanine,b) in the sublesion area of WT and S100A4−/−A/Sn mice after TBI. Number of animals,n=8/8 (WT/S100A4−/−), from two independent experiments, two-tailedt-test. (c–e) Neuronal death (c), oxidative stress (d) and expression of MTI+II (e) in the hippocampus of WT and S100A4−/−A/Sn mice after KA administration (20 mg kg−1). Inc,d,n=8/11, ine,n=9/12 andn=4/4 (intact). Two-tailedt-test (c,d) or two-way ANOVA (e). No TUNEL or 8-oxoguanine staining was detected in the intact brains. (a–e) Results are expressed as means±s.e.m. *P<0.05; **P<0.01; ***P<0.001. Scale bars, 50 μm (a–c), 500 μm (e). KO, knockout. Figure 2: S100A4 deficiency exacerbates brain injury. ( a , b ) Neuronal death (TdT-mediated dUTP nick end labeling (TUNEL), a ) and oxidative stress (8-oxoguanine, b ) in the sublesion area of WT and S100A4 −/− A/Sn mice after TBI. Number of animals, n =8/8 (WT/S100A4 −/− ), from two independent experiments, two-tailed t -test. ( c – e ) Neuronal death ( c ), oxidative stress ( d ) and expression of MTI+II ( e ) in the hippocampus of WT and S100A4 −/− A/Sn mice after KA administration (20 mg kg −1 ). In c , d , n =8/11, in e , n =9/12 and n =4/4 (intact). Two-tailed t -test ( c , d ) or two-way ANOVA ( e ). No TUNEL or 8-oxoguanine staining was detected in the intact brains. ( a – e ) Results are expressed as means±s.e.m. * P <0.05; ** P <0.01; *** P <0.001. Scale bars, 50 μm ( a – c ), 500 μm ( e ). KO, knockout. Full size image We next examined the effect of S100A4 deficiency in the mouse model of brain excitotoxicity. The KA-treated WT and S100A4 −/− mice had similar seizure profiles, most likely because the 2-h seizure recording period was insufficient for S100A4 upregulation. However, after 48 h, S100A4 −/− mice exhibited much more profound neuronal death in the hippocampus ( Fig. 2c , cell identity confirmed in Supplementary Fig. S1e ). Similar to the TBI model, it was paralleled by an increased number of neurons undergoing oxidative stress ( Fig. 2d ). In both models, no effect of S100A4 knockout was observed on reactive astrogliosis (GFAP staining), axonal or oligodendrocyte pathology (NF-200 or tau-1), or neuronal plasticity (GAP-43). Similarly, even though S100A4 has previously been shown to regulate macrophage chemotaxis [32] and thus it might affect post-traumatic inflammation, we did not find difference in the number of microglia/microphages in the sublesion zone (lectin staining). We speculated that S100A4 might also act indirectly by upregulating other neuroprotective proteins. Metallothionein I+II (MTI+II) is a major releasable neuroprotectant, similar to S100A4 found in astroglia and overexpressed in the excitotoxic hippocampus [33] , [34] . Strengthening the similarity, genetic deletion of MTI+II enhances neurodegeneration and oxidative stress in the excitotoxicity model [33] . We investigated a possible link between the S100A4 and MTI+II expression and found that the KA-induced MTI+II upregulation was markedly lower in the S100A4 −/− mice, with the difference most pronounced in the hippocampal CA1 region ( Fig. 2e ). MTI+II immunoreactivity was also increased in WM of WT animals both after KA treatment (injured/intact, 6.4±1.4% versus 2.4±0.2%) and after cryogenic brain trauma (ipsilateral injured/sham, 4.8±1.9% versus 2.5±0.4%). However, no effect of S100A4 deficiency on MTI+II expression in WM was observed in either model, suggesting that the S100A4-mediated MTI+II upregulation might be region-specific. Indeed, the basic levels of MTI+II in WM and hippocampus of control animals were markedly different (2.5±0.4% in WM versus 0.55±0.07 or 0.71±0.07% in CA1/CA3) indicating that different cell types and mechanisms could be involved in the MTI+II upregulation in these regions. Identification of neurotrophic motifs in the S100A4 sequence Several S100 proteins (S100B, S100A4, S100A12) affect neuritogenesis and/or survival of primary neurons [2] . Although S100B and S100A12 signal through the RAGE [9] , the neurotrophic activity of S100A4 appears independent of it [19] . We therefore reasoned that S100 proteins may have both homologous (‘common’) and specific (‘unique’) motifs conferring their effects. To explore this possibility, we generated synthetic peptides covering the sequences of S100A4 and S100A12 ( Supplementary Fig. S2a ), and tested them in rat hippocampal neurons, where both proteins act as trophic factors [2] . One peptide from S100A12 (H3A12) and two peptides from S100A4 (H3 and H6) mimicked neuritogenic effect of their ‘parent’ proteins ( Fig. 3a ). Interestingly, H3A12 and H3 corresponded to homologous and structurally similar regions of S100A12 and S100A4 ( Fig. 3a , blue, ‘common’ neuritogenic motif). However, H6 belonged to the C-terminus of S100A4 with little homology to other S100 proteins ( Fig. 3b , red, ‘unique’ neuritogenic motif). Both H3 and H6, as well as S100A4, were also neuritogenic in mouse hippocampal neurons ( Supplementary Fig. S2b ). Treatment of neurons with mutated versions of H3 or H6 ( Supplementary Fig. S2c,d ) showed that aa 89, 90 and 99–101 were important for neurite outgrowth, consistent with the previous data [35] involving the C-terminal residues (96–101) in biological effects of S100A4. Notably, both H3 and H6 in vitro activated messengers involved in S100A4-induced signalling [11] (Akt, ERK1/2 (extracellular signal-regulated kinase 1) and CREB (cAMP response element-binding), Fig. 3c ) and were neuroprotective in the models of oxidative stress ( Fig. 3d ) and KA excitotoxicity ( Fig. 3e ). The pro-survival effect of S100A4 and its peptide mimetics was decreased by pharmacological inhibition of the ERK1/2 pathway ( Fig. 3f ) and nearly abolished by blocking of Akt ( Fig. 3g ). Moreover, H3 and H6 crossed the blood–brain barrier when administered systemically ( Fig. 3h ), suggesting that they could be used as S100A4 mimetics to study its function in the brain. 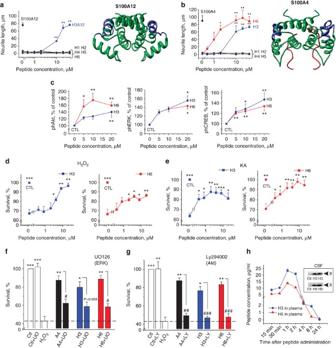Figure 3: Identification of neurotrophic motifs in S100A4. (a,b) S100-derived peptides were tested for their neurotrophic activity. One neuritogenic motif was found in the S100A12 sequence (H3A12,a), and two motifs in the S100A4 sequence (H3, H6,b). As positive controls, the respective recombinant proteins (5 μM) were used. ANOVA versus unstimulated cultures, four independent experiments. (a,b, right) Neuritogenic motifs of S100A12 and S100A4 mapped on 3D structures of the respective proteins (PDB:2WCE and 1M31). (c) The H3 and H6 peptides increase phosphorylation of messengers involved in S100A4-induced signalling, Akt, ERK and CREB, assessed by phosphospecific antibody cell-based ELISA and expressed relative to unstimulated controls (CTL). ANOVA versus CTL, five independent experiments. (d,e) H3 and H6 protect neurons from H2O2- (d) and KA- (e) induced death. CTL (100%), the survival rate in the untreated controls. ANOVA versus cultures treated with H2O2or KA only, four to five independent experiments. (f,g) Pharmacological blockers of mitogen-activated protein kinase (UO126, 20 μM,f) or Akt (LY294002, 20 μM,g) decrease the pro-survival effect of S100A4, H3 and H6 in the H2O2-treated neurons. Inhibitors alone (CTL+UO, CTL+LY) have no effect. CTL (100%), the survival rate in the untreated controls. S100A4, H3 and H6 are used at 20 μM. *versus H2O2only- treated cells; #, versus H2O2- and S100A4- or peptide-treated cells, two-way ANOVA, four independent experiments. (h) Plasma concentration time-course of H3 and H6 and determination of the peptides in cerebrospinal fluid (CSF) 1 h after a single subcutaneous administration to rats (10 mg kg−1). (a–h) Results are expressed as means±s.e.m. *,#P<0.05; **,##P<0.01; ***,###P<0.001. KO, knockout. Figure 3: Identification of neurotrophic motifs in S100A4. ( a , b ) S100-derived peptides were tested for their neurotrophic activity. One neuritogenic motif was found in the S100A12 sequence (H3A12, a ), and two motifs in the S100A4 sequence (H3, H6, b ). As positive controls, the respective recombinant proteins (5 μM) were used. ANOVA versus unstimulated cultures, four independent experiments. ( a , b , right) Neuritogenic motifs of S100A12 and S100A4 mapped on 3D structures of the respective proteins (PDB:2WCE and 1M31). ( c ) The H3 and H6 peptides increase phosphorylation of messengers involved in S100A4-induced signalling, Akt, ERK and CREB, assessed by phosphospecific antibody cell-based ELISA and expressed relative to unstimulated controls (CTL). ANOVA versus CTL, five independent experiments. ( d , e ) H3 and H6 protect neurons from H 2 O 2 - ( d ) and KA- ( e ) induced death. CTL (100%), the survival rate in the untreated controls. ANOVA versus cultures treated with H 2 O 2 or KA only, four to five independent experiments. ( f , g ) Pharmacological blockers of mitogen-activated protein kinase (UO126, 20 μM, f ) or Akt (LY294002, 20 μM, g ) decrease the pro-survival effect of S100A4, H3 and H6 in the H 2 O 2 -treated neurons. Inhibitors alone (CTL+UO, CTL+LY) have no effect. CTL (100%), the survival rate in the untreated controls. S100A4, H3 and H6 are used at 20 μM. *versus H 2 O 2 only- treated cells; #, versus H 2 O 2 - and S100A4- or peptide-treated cells, two-way ANOVA, four independent experiments. ( h ) Plasma concentration time-course of H3 and H6 and determination of the peptides in cerebrospinal fluid (CSF) 1 h after a single subcutaneous administration to rats (10 mg kg −1 ). ( a – h ) Results are expressed as means±s.e.m. * ,# P <0.05; ** ,## P <0.01; *** ,### P <0.001. KO, knockout. Full size image H3 and H6 peptides protect neurons in brain injury If S100A4 is neuroprotective, mimicking its functions in vivo should improve neuronal survival after brain injury. We employed the H3 and H6 peptides as tools to test this prediction. Following TBI in rats, S100A4 was overexpressed in WM and, interestingly, further upregulated by H6 contralaterally to the damage ( Fig. 4a ), suggesting that the post-traumatic S100A4 levels may also be regulated by an autocrine mechanism. In line with this, similar results were obtained in vitro , where S100A4 mRNA levels in the control astrocytes were not affected by extracellular S100A4 or H6, but in cells subjected to oxidative stress, S100A4 mRNA was upregulated by S100A4, and similar tendency was observed for H6 ( Fig. 4b ). 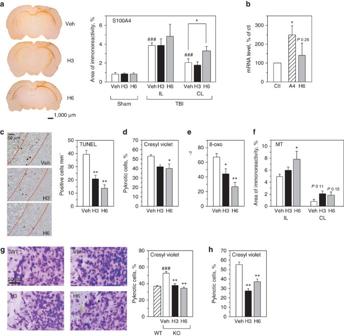Figure 4: S100A4 mimetics protect neurons in TBI (a) S100A4 expression in WM ipsi- (IL) and contralateral (CL) to TBI. Two-way ANOVA, *, versus CL Veh; #, versus Sham Veh. (b) Quantitative reverse transcription–PCR analysis of S100A4 mRNA levels in mouse hippocampal astrocytes subjected to oxidative stress (40 μM H2O2) and treated with S100A4 or the H6-peptide (both 20 μM). Ctl, H2O2only-treated cultures, set to 100%. Pairedt-test from three experiments, two reproductions each. (c,d) apoptotic cell death (c) and neurodegeneration (d, cresyl violet staining) in the sublesion area in vehicle-, H3- and H6-treated rats 96 h post injury. Number of animals (Veh/H3/H6),n=4/5/5 (a,d),n=7/8/8 (c). Sham-operated rats (a),n=5/3/4. (e,f) Oxidative stress (e, 8-oxoguanine, sublesion area) and MTI+II expression (f, WM) after TBI.n=7/6/6. (g) Neurodegeneration in the sublesion area of WT and S100A4−/−A/Sn mice treated with Veh, H3 or H6 and subjected to TBI. Left, representative images; right, quantification, cresyl violet staining,n=7/7/7. (h) Neurodegeneration in the sublesion area of C57BL/6j mice treated with Veh, H3 or H6 after induction of TBI,n=7/7/7. (c–h) ANOVA versus Veh. No TdT-mediated dUTP nick end labeling (TUNEL)-, 8-oxoguanine-, MTI+II-positive cells or damaged neurons (cresyl violet staining) were detected in shams. (a–h) Results are expressed as means±s.e.m. *,#P<0.05; **,##P<0.01; ***,###P<0.001. Scale bars, 1,000 μm (a), 50 μm (c,g). Figure 4: S100A4 mimetics protect neurons in TBI ( a ) S100A4 expression in WM ipsi- (IL) and contralateral (CL) to TBI. Two-way ANOVA, *, versus CL Veh; #, versus Sham Veh. ( b ) Quantitative reverse transcription–PCR analysis of S100A4 mRNA levels in mouse hippocampal astrocytes subjected to oxidative stress (40 μM H 2 O 2 ) and treated with S100A4 or the H6-peptide (both 20 μM). Ctl, H 2 O 2 only-treated cultures, set to 100%. Paired t -test from three experiments, two reproductions each. ( c , d ) apoptotic cell death ( c ) and neurodegeneration ( d , cresyl violet staining) in the sublesion area in vehicle-, H3- and H6-treated rats 96 h post injury. Number of animals (Veh/H3/H6), n =4/5/5 ( a , d ), n =7/8/8 ( c ). Sham-operated rats ( a ), n =5/3/4. ( e , f ) Oxidative stress ( e , 8-oxoguanine, sublesion area) and MTI+II expression ( f , WM) after TBI. n =7/6/6. ( g ) Neurodegeneration in the sublesion area of WT and S100A4 −/− A/Sn mice treated with Veh, H3 or H6 and subjected to TBI. Left, representative images; right, quantification, cresyl violet staining, n =7/7/7. ( h ) Neurodegeneration in the sublesion area of C57BL/6j mice treated with Veh, H3 or H6 after induction of TBI, n =7/7/7. ( c – h ) ANOVA versus Veh. No TdT-mediated dUTP nick end labeling (TUNEL)-, 8-oxoguanine-, MTI+II-positive cells or damaged neurons (cresyl violet staining) were detected in shams. ( a – h ) Results are expressed as means±s.e.m. * ,# P <0.05; ** ,## P <0.01; *** ,### P <0.001. Scale bars, 1,000 μm ( a ), 50 μm ( c , g ). Full size image Corroborating the effects of S100A4 knockout in TBI, both peptides reduced apoptotic neuronal death in the sublesion area by 50% (H3) or 70% (H6) ( Fig. 4c ), improved neuronal survival ( Fig. 4d and Supplementary Fig S3a ) and robustly protected cells against oxidative stress ( Fig. 4e ). We also tested how the peptides affect the expression of MTI+II after TBI. In accordance with the previous data [33] , MTI+II was not detectable in the brains of sham-operated rats, but was induced in WM following trauma ( Fig. 4f ). Treatment with H6 significantly increased post-traumatic upregulation of MTI+II in WM adjacent to the lesion, and both peptides tended to also upregulate MTI+II contralaterally ( Fig. 4f ). We next tested whether S100A4 mimetics can substitute for its functions in S100A4-deficient animals. Confirming our previous findings ( Fig. 2a ), the S100A4 knockout mice were more susceptible to brain trauma than their WT littermates ( Fig. 4g and Supplementary Fig. S3b ). Both H3 and H6 decreased neuronal loss in S100A4 −/− animals to the WT level, indicating that the peptides exerted direct neuronal effect mimicking that of extracellular S100A4 ( Fig. 4g and Supplementary Fig. S3b ). To address the therapeutic potential of S100A4 peptides in a clinically relevant experimental setup, we treated mice with H3 or H6 after induction of TBI. When first injected 2 h after brain trauma, both peptides reduced the delayed neuronal death nearly two-fold ( Fig. 4h and Supplementary Fig. S3c ), suggesting that they could be useful means for developing neuroprotective therapies. The S100A4 mimetics were also beneficial in the excitotoxicity model. H3- or H6-treated mice had fewer seizure episodes after KA administration (20 mg kg −1 , Fig. 5a , stages 1–4). Summarized by severity, H3 and H6 markedly attenuated both low-grade and high-grade seizures ( Fig. 5b ). The peptides were also protective against more severe excitotoxicity induced by a high KA dose (30 mg kg −1 ), which caused 60% mortality in the vehicle group. In this experimental setup, mice receiving the peptides had almost two-fold higher survival rates ( Fig. 5c ). Accordingly, the peptide-treated mice had lower neurodegeneration in the hippocampus 24 h after KA administration (20 mg kg −1 ), reaching significance in the H6-receiving group ( Fig. 5d ) and exhibited an increased hippocampal expression of MTI+II ( Fig. 5e ). Thus, the effects of the S100A4 mimetics in the two models of brain injury supported the neuroprotective function of S100A4 in vivo and suggested that the S100A4-induced upregulation of MTI+II is one of the mechanisms behind it. 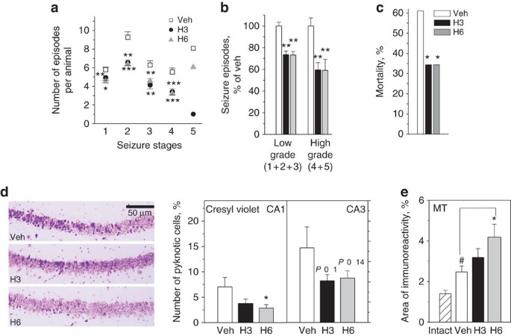Figure 5: S100A4 mimetics are neuroprotective against KA-induced excitotoxicity. (a,b) H3 and H6 ameliorate KA-induced seizures in C57BL/6j mice (a), summarized by severity inb. Seizure episodes are scored 1–5 by increasing severity as described in the Methods.n=14/14/14, ANOVA versus Veh. (c) H3 and H6 decrease KA-induced mortality.n=31/31/31, Fisher’s exact test versus Veh. (a–c), four independent experiments. (d) Neurodegeneration in the hippocampus 24 h after KA administration (20 mg kg−1), cresyl violet staining. Virtually no pyknotic cells were detected in the intact hippocampi (not depicted). Scale bar, 50 μm.n=8/8/8, ANOVA versus Veh. (e) MTI+II expression in the hippocampus. Intact/Veh/H3/H6,n=5/6/4/6, *ANOVA versus Veh; # two-tailedt-test versus Intact. (a,b,d,e) Results are expressed as means±s.e.m. *,#P<0.05; **,##P<0.01; ***,###P<0.001. Figure 5: S100A4 mimetics are neuroprotective against KA-induced excitotoxicity. ( a , b ) H3 and H6 ameliorate KA-induced seizures in C57BL/6j mice ( a ), summarized by severity in b . Seizure episodes are scored 1–5 by increasing severity as described in the Methods. n =14/14/14, ANOVA versus Veh. ( c ) H3 and H6 decrease KA-induced mortality. n =31/31/31, Fisher’s exact test versus Veh. ( a – c ), four independent experiments. ( d ) Neurodegeneration in the hippocampus 24 h after KA administration (20 mg kg −1 ), cresyl violet staining. Virtually no pyknotic cells were detected in the intact hippocampi (not depicted). Scale bar, 50 μm. n =8/8/8, ANOVA versus Veh. ( e ) MTI+II expression in the hippocampus. Intact/Veh/H3/H6, n =5/6/4/6, *ANOVA versus Veh; # two-tailed t -test versus Intact. ( a , b , d , e ) Results are expressed as means±s.e.m. * ,# P <0.05; ** ,## P <0.01; *** ,### P <0.001. Full size image S100A4 protects neurons via JAK/STAT and the IL-10 receptor To identify candidate receptors mediating the pro-survival effect of S100A4, we pulled down putative S100A4 targets from neuronal lysates using the S100A4-specific H6-motif as bait. The pull-down yielded a number of candidate-binding partners for S100A4, which were identified by liquid chromatography–mass spectrometry ( Fig. 6a ). Focusing on plasma membrane targets known to activate pro-survival signalling, we chose the interleukin-10 receptor-α (IL-10R) for further testing. 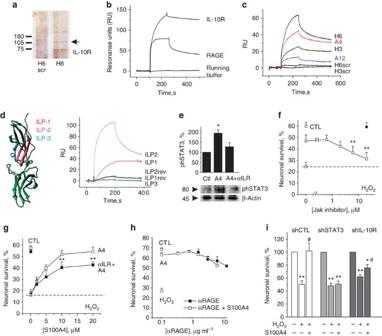Figure 6: S100A4 protects neurons via JAK/Stat3 and partially IL-10Rα. (a) Silver staining of putative binding partners of S100A4 pulled down from neuronal lysates with the H6 peptide as bait and scrambled H6 (H6scr) as a negative control. IL-10Rα (identified by liquid chromatography–mass spectrometry). (b) SPR binding of IL-10R (1 μM) to S100A4, with RAGE as a positive control. (c) SPR binding of recombinant S100A4, S100A12 (0.5 μM each), H3, H6 or their scrambled (scr) versions (2 μM each) to IL-10R. (d) Putative S100A4-interacting motifs (ILP1-3) in IL-10R mapped on its 3D structure (PDB:1Y6K) and SPR binding of the ILP1-3 peptides and their reversed versions, ILPrev1-3 (2.5 μM each), to S100A4. (a–d) are representative of two to three independent experiments. (e) S100A4-induced phosphorylation of STAT3 in neurons (A4, 20 μM) is decreased by IL-10R antibodies (αILR). (f,g) Pharmacological blocker of JAK (f) or inhibitory IL-10R antibodies (αILR,g) decrease the pro-survival effect of S100A4 in the H2O2-treated neurons. The JAK inhibitor (f, ■) or anti-IL-10R antibody (g, ■) alone have no effect. CTL, untreated controls. Inf, S100A4 is used at 20 μM. (h) Inhibitory RAGE antibodies (αRAGE) do not reduce the pro-survival effect of S100A4 (20 μM) in the H2O2-treated neurons. CTL, untreated controls; (■), the αRAGE antibodies alone applied to CTL, two-way ANOVA. (i) Knockdown of STAT3 or IL-10R reduces S100A4-induced neuroprotection (A4, 20 μM). For each shRNA, the survival of transfected neurons was normalized to untreated controls (100%). *, versus untreated; #, versus H2O2only-treated cells. (e–i) are data from four to five independent experiments, results are expressed as means±s.e.m. ANOVA (e,f) or two-way ANOVA (g–i), *,#P<0.05; **,##P<0.01. Figure 6: S100A4 protects neurons via JAK/Stat3 and partially IL-10Rα. ( a ) Silver staining of putative binding partners of S100A4 pulled down from neuronal lysates with the H6 peptide as bait and scrambled H6 (H6scr) as a negative control. IL-10Rα (identified by liquid chromatography–mass spectrometry). ( b ) SPR binding of IL-10R (1 μM) to S100A4, with RAGE as a positive control. ( c ) SPR binding of recombinant S100A4, S100A12 (0.5 μM each), H3, H6 or their scrambled (scr) versions (2 μM each) to IL-10R. ( d ) Putative S100A4-interacting motifs (ILP1-3) in IL-10R mapped on its 3D structure (PDB:1Y6K) and SPR binding of the ILP1-3 peptides and their reversed versions, ILPrev1-3 (2.5 μM each), to S100A4. ( a – d ) are representative of two to three independent experiments. ( e ) S100A4-induced phosphorylation of STAT3 in neurons (A4, 20 μM) is decreased by IL-10R antibodies (αILR). ( f , g ) Pharmacological blocker of JAK ( f ) or inhibitory IL-10R antibodies (αILR, g ) decrease the pro-survival effect of S100A4 in the H 2 O 2 -treated neurons. The JAK inhibitor ( f , ■) or anti-IL-10R antibody ( g , ■) alone have no effect. CTL, untreated controls. In f , S100A4 is used at 20 μM. ( h ) Inhibitory RAGE antibodies (αRAGE) do not reduce the pro-survival effect of S100A4 (20 μM) in the H 2 O 2 -treated neurons. CTL, untreated controls; (■), the αRAGE antibodies alone applied to CTL, two-way ANOVA. ( i ) Knockdown of STAT3 or IL-10R reduces S100A4-induced neuroprotection (A4, 20 μM). For each shRNA, the survival of transfected neurons was normalized to untreated controls (100%). *, versus untreated; #, versus H 2 O 2 only-treated cells. ( e – i ) are data from four to five independent experiments, results are expressed as means±s.e.m. ANOVA ( e , f ) or two-way ANOVA ( g – i ), * ,# P <0.05; ** ,## P <0.01. Full size image We examined whether IL-10R directly interacted with S100A4 by surface plasmon resonance (SPR) analysis, using RAGE, known to bind S100A4 (refs 9 , 19 ), as a positive control ( Fig. 6b ). IL-10R bound to immobilized S100A4 with the affinity Kd=5.7±2.1 nM, as determined based on binding kinetics ( Fig. 6b and Supplementary Fig. S4a ). Moreover, S100A4 added extracellularly co-migrated with IL-10R overexpressed in HEK-293 cells after chemical cross-linking at the cell surface ( Supplementary Fig. S4b ). In the reversed SPR experiment, IL-10R, immobilized on a sensor chip, interacted with soluble S100A4, the H3- or the H6-peptides, but not with the scrambled peptide versions ( Fig. 6c ). Thus, both functional motifs of S100A4 were likely involved in its interaction with IL-10R. Furthermore, we found that the extracellular module of IL-10R contains four motifs homologous to the motifs in the extracellular part of the S100A4 binding partner RAGE ( Supplementary Fig. S4c , ILP1-4). Synthetic peptides encompassing ILP1 and ILP2, but not ILP3, sequence-specifically bound to the immobilized S100A4 protein ( Fig. 6d ), thus likely constituting the IL-10R binding site for S100A4. IL-10R is expressed in the brain [36] and signals through the JAK/STAT3 pathway [37] . Its ligand, IL-10, promotes neuronal survival in several models of brain and spine injury (ref. 38 and references therein). Accordingly, extracellular S100A4 induced STAT3 phosphorylation in neurons, which was diminished by inhibitory IL-10R antibodies ( Fig. 6e ). Moreover, pharmacological blockade of JAK reduced S100A4-induced survival in the in vitro model of oxidative stress ( Fig. 6f ). Antibodies to IL-10R had similar effect ( Fig. 6g ), but inhibition was only partial, suggesting that additional receptors may be involved in neuroprotection by S100A4. One of such receptors could potentially be RAGE, a common S100-binding partner. However, neutralizing antibodies to RAGE previously shown to inhibit RAGE-mediated effects in neurons [39] had no effect on the S100A4-induced survival ( Fig. 6h ). To confirm our results, we knocked down the expression of IL-10R or STAT3 in neurons and subjected these cultures to oxidative stress in vitro . We found that the pro-survival effect of S100A4 was reduced by STAT3 or, to a lesser extent, IL-10R ablation ( Fig. 6i ). Combined, these findings corroborated the hypothesis that both IL-10R and STAT3 are involved in S100A4-induced neuronal survival. In this study, we show a novel neuroprotective role for the cancer-related S100A4 protein and introduce the S100 family as a potential class of neuroactive factors. In vivo data on the role of S100 proteins in brain damage are only available for S100B and remain controversial: administered at low doses, S100B improves TBI outcome, but its overexpression exacerbates brain trauma [7] . This finding was related to the dual effect of S100B in vitro , where it was neuroprotective at low but detrimental at higher concentrations [7] . For S100A4, we only found a neuroprotective, but no cytotoxic effect, suggesting that the two proteins act through separate mechanisms. First, extracellular S100A4 may rescue neurons via the IL-10R/JAK/STAT3 pathway, which upregulates multiple antioxidant enzymes and neuroprotective genes in neural cells [40] , [41] . S100A4 may also activate the IL-10R/Akt signalling cascade, which was previously shown to mediate the IL-10-induced neuronal survival [42] , [43] . However, our data indicate that additional receptor(s) are involved in S100A4-induced neuroprotection. Interesting candidates may be ErbB receptors, which, as we have recently shown, can be indirectly activated by extracellular S100A4 (ref. 44 ) and trigger signalling through JAK/STAT [45] , ERK and Akt [46] , the messengers involved in the S100A4-induced survival ( Fig. 3f ). Thus, biological effects of S100A4 in the brain are likely mediated by multiple plasma membrane targets, with their relative importance defined by the expression pattern and physiological settings. Detailed characterization and in vivo validation of this ‘S100A4 receptor toolbox’ is a challenging direction for future studies. As a second neuroprotective mechanism, S100A4 overexpression in astrocytes may regulate other glia-derived factors, such as the releasable neuroprotectant MTI+II, as demonstrated here. MTI+II has numerous beneficial effects in the injured CNS acting as a reactive oxygen species scavenger intracellularly and triggering pro-survival signalling via cell surface receptors when secreted [33] , [47] . These MTI+II activities were reported to decrease secondary neuronal damage and post-traumatic inflammation and to promote tissue repair [33] , thus likely amplifying the direct neuroprotective effect of S100A4. Moreover, our results raise the intriguing possibility that S100A4 and MTI+II could interplay in other pathologies, for example developing tumours, where both proteins are overexpressed and functionally important [10] , [48] . This study also provides a rationale for exploring pharmacological means to modulate S100A4 expression and functions in the injured brain. A promising approach may be designing small mimetic peptides encompassing biologically active motifs of S100A4, as shown here. Such mimetics can be easily synthesized, administered and modified to provide maximal therapeutic effect. Moreover, because they represent relatively short sequences isolated to confer a specific protein’s function, these peptides are less likely to have side effects than the full-length protein. Importantly, our results indicate that other S100 proteins may also be of high interest as potential therapeutic targets in CNS. Indeed, the presence of two neuroactive motifs in the S100A4 molecule, one of which is ‘shared’ within the family, suggests that several S100 proteins may have yet undiscovered functions in the nervous system. Some of the S100 activities in the brain may be defined by their common target, RAGE, but accumulating evidence suggests that RAGE is not a sole receptor for S100 [19] , [44] , [49] , presenting a fascinating field for future research. In summary, this is to our knowledge the first report establishing S100A4 as a neuroprotective factor in vivo . Our data extend the view of S100A4 from tumour promoter to a multifunctional protein, whose effects strongly depend on the physiological context. Because S100A4 is associated with glia, its role may be even more prominent in the human brain where the astrocyte/neuron ratio is higher than in rodents [50] . The general antioxidative and antiexcitotoxic effects of S100A4 suggest that it can protect cells in many types of neurodegeneration, thereby emerging as an interesting therapeutic target. Moreover, the entire S100 protein family may be a previously underrated, but a potentially important factor in CNS disorders. Human brain tissue Pericontusional human cerebral samples were obtained from the tissue bank of Hospital Universitario Marqués de Valdecilla, Santander, Spain. Tissue specimens were retrieved from patients with cortical brain trauma undergoing emergency craniotomy as described in Minambres et al . [51] Samples of intact human brain were from Capital Biosciences (Rockville, MD, USA). All experiments with human tissues complied with institutional regulations. Animals The animal protocols were approved by the Danish Animal Experiments Inspectorate. Male Wistar rats (6 weeks, 100–150 g) and female C57BL/6j mice (11 weeks, 25–30 g) were from Taconic (Denmark). S100A4 −/− mice on an A/Sn background (8–10 wks) were generated and genotyped as described in El Naaman et al . [26] , and were not phenotypically different from WT A/Sn mice, used as controls. Peptides and recombinant proteins Peptides (see Supplementary Figs S2a and S4c for sequences) were synthesized as tetramers composed of four monomers coupled to a lysine backbone (Schafer-N, Denmark). Tetramerization was previously found to be necessary for the neuritogenic activity of S100A4 (ref. 11 ). When applicable, peptide biotinylation was performed (Schafer-N, 90% purity). Recombinant S100A4 and S100A12 were produced as described in Novitskaya et al . [11] and Mikkelsen et al . [52] Neuronal survival assay Rat hippocampal neurons (E19) were prepared according to Soroka et al . [53] After seven days in vitro (DIV), neurons were treated with S100A4, H3 or H6 for 1 h followed by KA (300 μM) or H2O2 (60 μM, both from Sigma). Inhibitory antibodies to IL-10R (R&D Systems) or the JAK inhibitor (Calbiochem) were added 30 min before S100A4. For knockdown experiments, neurons were electroporated before plating [54] with 2 μg plasmid DNA encoding shRNA for rat IL-10R, STAT3 or nontargeting shRNA (OriGene, Rockville, MD, USA), all cloned in pGFP plasmid. After three DIV, neurons were consecutively treated with S100A4 and H 2 O 2 as described above, further cultured for 24 h, fixed and stained with Hoechst 33258 (Invitrogen). Analysis of neuronal survival was performed as previously described [54] , [55] . To quantify the numbers of surviving transfected neurons, the cells were counterstained for green fluorescent protein. Neurite outgrowth and phosphorylation assays Hippocampal neurons were stimulated with peptides, grown for 24 h and stained with Coomassie Blue R250. Neurite outgrowth was evaluated as described in Soroka et al . [53] Phosphorylation of Akt, CREB and ERK was determined by phosphospecific antibody cell-based enzyme-linked immunosorbent assay (ELISA) as the ratio of phosphorylated to total protein [56] . Cryogenic lesion A focal cryolesion [24] , [25] was produced on the surface of the right brain hemisphere by placing a pellet of dry ice onto the skull for 60 s (rats) or for 30 s (mice). The injured area was localized over the sensorimotor cortex (anterior/posterior/lateral edges, mm: +1.0/−2.0/3.0 for mice and +1.0/−3.0/4.0 for rats). Peptides (10 mg kg −1 ) were administered subcutaneously using the following regiments: rats ( Fig. 4c–f )—24 h before, 24 and 72 h after surgery; A/Sn WT and S100A4 −/− mice ( Fig. 4g )—24 h before, 24 and 48 h after surgery; C57BL/6j mice ( Fig. 4h )–2, 24, and 48 h after surgery. Animals were killed 72 h (mice) or 96 h (rats) after surgery. KA-induced excitotoxicity C57BL/6j male mice were injected with vehicle or peptides 48, 24 and 2 h before KA treatment (i.p.). Two sets of experiments were performed to induce either low-grade seizures (20 mg kg −1 KA) or high-grade seizures and mortality (30 mg kg −1 KA) [54] , [57] . In another set of experiments, WT and S100A4 −/− A/Sn male mice were used, receiving 20 mg kg −1 KA only. Seizure activity was assessed for 2 h following KA administration [54] , [57] . Mice were killed 24 or 48 h after KA administration. Histology Animal perfusion and brain processing were performed as previously described [24] . Hippocampal morphology was assessed stereologically using 30 μm coronal sections (six per animal) stained with 0.5% cresyl violet (Nissl staining). In all experiments, numbers of pyknotic (P) and viable (V) neurons were quantified, and the percentage of pyknotic cells was calculated as P/(P+V) × 100%. In the KA excitotoxicity model (20 mg kg −1 ), cell death in the hippocampus was <10% of the total population, and thus the number of viable cells did not change significantly. Therefore, only the numbers of pyknotic cells were presented. In situ DNA fragmentation was evaluated on the 7 μm coronal sections using a TUNEL kit (Calbiochem). To label microglia/macrophages, biotinylated tomato lectin (1:500, Sigma) was used. Immunohistochemistry was performed on 7 μm coronal sections (three per animal) as described in Klementiev et al . [24] We used the following primary antibodies: anti-GAP-43 (1:400; Chemicon), anti-GFAP (1:500; DakoCytomation), anti-human S100A4 (1:200) [14] , anti-mouse S100A4 (1:1,000) [16] , [26] , anti-MTI+II (1:250, DakoCytomation), anti-8-oxoguanine (1:1,000, Millipore), anti-NF-200 (1:1,000, Sigma), anti-tau1 (1:4,000, Millipore) and anti-NeuN (1:250, Chemicon), followed by biotin-conjugated (Sigma) or Alexa Fluor-conjugated (Invitrogen) secondary antibodies. Negative controls were prepared identically, but the primary antibody was omitted. Autofluorescence in the human brain samples was reduced by ultraviolet irradiation combined with NaBH 4 and Sudan Black treatments [58] . Microscopy and morphometric analysis Images were acquired using an Olympus BX-51 microscope and the Visiopharm Integrator System software (Visiopharm). Quantifications were performed in the hippocampus (KA excitotoxicity model) or sublesion area (TBI). Sections (3–6 per animal) were analysed using the computer-assisted Stereological Toolbox programme with unbiased sampling (CAST-2, Olympus) by a researcher blinded to treatment. Immunoreactivity area was quantified using the PrAverB software (Protein Laboratory, University of Copenhagen, Denmark). Determination of H3 and H6 concentrations in plasma The study was performed with biotin-labelled H3 and H6, possessing similar neuritogenic activity to the unlabelled peptides. The peptides (10 mg kg −1 ) were administered to Wistar rats subcutaneously. Blood samples and cerebrospinal fluid were collected, and peptide concentrations in plasma were measured using a competitive ELISA ( n =5–7 animals for each time point, two independent determinations) [24] , [54] . Biotinylated peptides in cerebrospinal fluid were detected by immunoblotting using HRP-conjugated streptavidin (1:1,000, Dako-Cytomation). S100A4 release from astrocytes Mouse hippocampal astrocytes (P1) were plated in poly- L -lysin-coated culture flasks and cultured in serum-supplemented DMEM. At 10 DIV, cells were replated into 24-well culture plates (Nunc), grown to confluence, and cultured for 2 further days in the Neurobasal Medium. Astrocytes were treated with H 2 O 2 for 2, 6 or 24 h, and samples of medium were collected. S100A4 concentrations in the samples were measured using a sandwich ELISA [16] ( n =6 experiments, two independent determinations) and normalized to protein levels in each sample. Samples showing lower (70–90% of average) cell counts due to cell death at a high H 2 O 2 concentration were designated as ‘damaged’ and processed as a separate group. Quantitative reverse transcription–PCR analysis of S100A4 expression Mouse hippocampal astrocytes (5 × 10 6 ) were seeded in 30 mm tissue culture dishes, grown to 80% confluency and treated with 10 μM S100A4 or H6 followed by 80 μM H 2 O 2 for 24 h. Total RNA preparation, quantitative reverse transcription–PCR and data analysis were performed as described previously [59] using following primers: S100A4_F: 5′-GGCAAGACCCTTGGAGGAGGC-3′; S100A4_R: 5′-GCTGTCCAAGTTGCTCAT-3′; GAPDH_F: 5′-AAGGTCATCCCAGAGCTGAACG-3′; GAPDH_R: 5′-CCTGCTTCACCACCTTCTTGAT-3′. All samples were run in duplicates. The relative levels of the PCR products in all samples were evaluated by the Pfaffl method [60] . Immunoblotting assay Neurons (3 × 10 6 cells) were grown for 4 h before treatment. Immunoblotting was performed as described previously [19] . Rabbit anti-phospho-STAT3 antibodies (1:1,000; Cell Signaling) or rabbit anti-β-actin (1:2,000; Sigma) were used. STAT3 phosphorylation was normalized to β-actin levels for each sample. Affinity chromatography The H6 peptide or its scrambled version, H6scr (2 mg each), were immobilized on CNBr-activated Sepharose 4B (Amersham). Packed H6 and H6scr columns were equilibrated in starting buffer (100 mM NaCl, 2 mM CaCl 2 , 10 mM HEPES, pH 7.3), and neuron lysates (5 × 10 7 cells) dissolved in the starting buffer were applied on each column. After washing, bound proteins were retrieved by incubating sepharose beads in SDS–PAGE loading buffer and separated by electrophoresis. The bands were visualized using the SilverQuest Silver Staining Kit (Invitrogen), excised and identified by liquid chromatography–mass spectrometry (Institute of Biochemistry and Biophysics, Warsaw, Poland). 3,3′-dithiobis(sulfosuccinimidylpropionate) cross-linking HEK-293 cells were grown in 10-cm petri dishes to confluency and transiently transfected with either empty vector or the Myc-conjugated IL-10R construct (OriGene). Twenty-four hours after transfection, cells were incubated with 10 μM S100A4 (1 h, 4 °C) followed by 10 mM thiol-cleavable cross-linker 3,3′-dithiobis (sulfosuccinimidylpropionate) (30 min, room temperature). Cross-linking was terminated by adding 50 mM Tris–Cl (pH 7.5, 15 min). The cells were lysed in the thiol-free lysis buffer, and the cross-linked proteins were resolved by SDS–PAGE followed by immunoblotting using antibodies against S100A4 (1:2,000) [26] and anti-Myc (1:1,000, OriGene) and IRDye secondary antibodies (Odyssey, Lincoln, Nebraska, USA). The bands were visualized using Odyssey CLX Infrared Imaging System (Odyssey). SPR analysis SPR experiments were performed using a BIAcore 2000 instrument (Biacore). To study ligand binding to S100 proteins, 2,000 resonance units of recombinant human S100A12, S100A4 or the human extracellular IL-10R/Fc chimera (R&D Systems) were immobilized covalently on a CM4 sensor chip (Biacore). Binding and data analysis were performed as described previously [19] . For each condition, two independent experiments were performed. Statistics Statistics was performed using Origin 6.1 software (OriginLab) and GraphPad Prism 4.0 (GraphPad) by two-tailed t -test, one-way analysis of variance (ANOVA) or two-way ANOVA with Tukey’s post-test to identify statistically significant groups. Leven’s test was used to assess the equality of variances in groups, Shapiro–Wilk was used as a data normality test and Fisher’s exact test was used to evaluate mortality. Results are expressed as means±s.e.m., * P <0.05; ** P <0.01; *** P <0.001. How to cite this article: Dmytriyeva, O. et al . The metastasis-promoting S100A4 protein confers neuroprotection in brain injury. Nat. Commun. 3:1197 doi: 10.1038/ncomms2202 (2012).